Femtosecond nonlinear ultrasonics in gold probed with ultrashort surface plasmons Fundamental interactions induced by lattice vibrations on ultrafast time scales have become increasingly important for modern nanoscience and technology. Experimental access to the physical properties of acoustic phonons in the terahertz-frequency range and over the entire Brillouin zone is crucial for understanding electric and thermal transport in solids and their compounds. Here we report on the generation and nonlinear propagation of giant (1 per cent) acoustic strain pulses in hybrid gold/cobalt bilayer structures probed with ultrafast surface plasmon interferometry. This new technique allows for unambiguous characterization of arbitrary ultrafast acoustic transients. The giant acoustic pulses experience substantial nonlinear reshaping after a propagation distance of only 100 nm in a crystalline gold layer. Excellent agreement with the Korteveg-de Vries model points to future quantitative nonlinear femtosecond terahertz-ultrasonics at the nano-scale in metals at room temperature. Investigations of nanometre-wavelength, terahertz-frequency acoustic phonons usually require sophisticated methods with high spatial resolution such as X-rays [1] , electrons [2] or far ultraviolet radiation [3] . In metals, measurements at visible or infrared wavelengths intrinsically bear the potential of nanometre spatial resolution due to the characteristic penetration depth (skin depth) of optical fields of ~10 nm. Time-resolved optical experiments in metal and semiconductor thin films [4] provide a detailed picture of the generation of picosecond acoustic pulses [5] . However, the detection capabilities in picosecond ultrasonics are generally limited by the largely unknown photo-elastic coefficients leading to complicated dynamics of strain-induced surface reflectivity, rendering the characterization of acoustic pulses extremely challenging [6] , [7] . Some of these difficulties have been circumvented by using a more straightforward beam deflection technique [8] or equivalent interferometric detection of transient surface deformations [9] . Nevertheless, the separation of geometrical and photo-elastic contributions to the optical phase still represents a problem. An even more complicated experimental geometry utilizing joint phase- and polarization-sensitive reflectivity measurements at oblique light incidence was theoretically proposed to solve this problem [10] . Inspired by the performance of the first acousto-plasmonic pump-probe experiments in Kretschmann geometry in 1988 (ref. 11 ) and the recent progress in lateral nanofabrication techniques in hybrid multilayer structures combined with quantitative nanoplasmonic measurements below the optical skin depth [12] , [13] , we have developed femtosecond surface plasmon interferometry [14] . The phase of surface plasmons propagating along the metal-dielectric interface is not sensitive to transient surface displacements, but is only affected by the strain-induced photo-elastic contribution [13] . As demonstrated below, this fact allows us to fully characterize ultrashort acoustic pulses in gold by monitoring transient modulations of the surface plasmon wave vector. Beyond these important metrological issues, recent studies have revealed the possibility to generate ultrashort acoustic pulses by magnetostriction [15] , to manipulate the magnetization in ferromagnetic semiconductors [16] , [17] and metals [18] by ultrashort strain pulses, and to use acoustic pulses to generate terahertz radiation [19] . These findings render the field of terahertz acoustics truly interdisciplinary. Pioneering investigations of nonlinear acoustic dynamics in dielectric crystals at low temperature [9] , [20] have revealed clear signatures of shock-front decay into a sequence of acoustic solitons after a propagation distance of hundreds of microns. Surprisingly, acoustic nonlinearities have never been investigated in metals, although they are used as sources of large-amplitude acoustic pulses for these experiments. In this article, we demonstrate optical generation of large-amplitude acoustic strain pulses in a hybrid gold/cobalt bilayer structure and we observe nonlinear acoustic propagation effects in gold at the nano-scale. Acousto-plasmonics in a hybrid Au–Co multilayer structure We perform quantitative measurements by plasmonic pump-probe interferometry with femtosecond time resolution [14] . 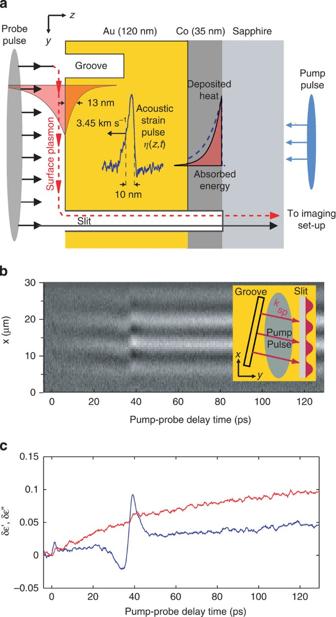Figure 1: Acousto-plasmonics in a hybrid gold–cobalt multilayer structure. (a) Schematic drawing of the acousto-plasmonic pump-probe experiment: surface plasmons propagating at the gold–air interface probe the reflection of acoustic pulses generated in the laser-heated cobalt transducer. (b) Measured acousto-plasmonic pump-probe interferogram showing a pronounced shift of the interference fringes upon reflection of an ultrashort acoustic pulse. The inset illustrates the geometry of the plasmonic slit-groove interferometer (see12,13,14for details). (c) Ultrafast dynamics of the real (red line) and imaginary (blue line) parts of the surface dielectric function extracted from the plasmonic interferogram. Panelsaandbare adapted from13. Figure 1a shows the experimental configuration of this technique adopted to study acousto-plasmonic effects. In contrast to most previous measurements performed with a single polycrystalline metal layer on a dielectric substrate, we use a Au/Co/sapphire structure with well-defined crystallographic orientation. A hybrid acousto-plasmonic 120 nm gold/35 nm cobalt/sapphire multilayer structure was manufactured by magnetron sputtering of a (111) gold layer on top of a hcp-cobalt film deposited on a (0001) sapphire substrate. The cobalt layer excited by an intense ultrashort laser pulse through the sapphire substrate serves as an efficient and ultrafast opto-acoustic transducer. Owing to strong electron-phonon relaxation on the time scale of 200–300 fs (ref. 21 ) and the short electron mean free path l e ~1 nm (ref. 22 ) in ferromagnetic materials, hot electron diffusion is much less efficient than in noble metals [23] . Therefore, the heat penetration depth only slightly exceeds the skin depth for pump light (typically by ~50%(ref. 5 )), see Fig. 1a . The laser-heated cobalt layer thermally expands and generates an ultrashort acoustic strain pulse propagating both into the gold layer and into the sapphire substrate. Excellent acoustic impedance matching between the three layers suppresses acoustic reflection at both the gold–cobalt and cobalt–sapphire interfaces (about 10%). As a consequence, the initial shape of a unipolar acoustic pulse follows the spatial profile of deposited heat in cobalt. The nonlinear dynamics of ultrashort acoustic pulses in sapphire have been addressed in detail before [9] , [20] . Here we focus on nonlinear acousto-plasmonic effects in a metal. Figure 1: Acousto-plasmonics in a hybrid gold–cobalt multilayer structure. ( a ) Schematic drawing of the acousto-plasmonic pump-probe experiment: surface plasmons propagating at the gold–air interface probe the reflection of acoustic pulses generated in the laser-heated cobalt transducer. ( b ) Measured acousto-plasmonic pump-probe interferogram showing a pronounced shift of the interference fringes upon reflection of an ultrashort acoustic pulse. The inset illustrates the geometry of the plasmonic slit-groove interferometer (see 12 , 13 , 14 for details). ( c ) Ultrafast dynamics of the real (red line) and imaginary (blue line) parts of the surface dielectric function extracted from the plasmonic interferogram. Panels a and b are adapted from [13] . Full size image The compressional acoustic pulse in gold creates a layer of higher ion density , which moves at the sound velocity c s =3.45 km s −1 in gold in the (111) direction. As the stationary charge separation between electrons and ions in a metal occurs only within the Debye radius r Debye ~10 −3 nm, the spatial profile of electron (charge) density n e ( z , t ) exactly follows the ionic one: n e ( z , t )= n i ( z , t ). At the probe photon energy of 1.55 eV of the probe pulses, the dielectric function ε m = ε ′+ iε ″=−24.8+1.5 i in gold is dominated by the free-carrier contribution with . An ultrashort acoustic strain pulse creates a time-dependent spatial profile of the dielectric function ε ′( z , t )= ε ′(1+ η ( z , t )) inside the metal, which modulates the surface plasmon wave vector , when the strain pulse arrives within the surface plasmon skin depth δ skin =13 nm at the gold–air interface: Figure 1b shows the experimental time-resolved plasmonic pump-probe interferogram. It depicts the pump-induced changes of optical properties at the gold–air interface captured by time-delayed surface plasmon probe pulses and recorded in optical transmission through the slit. Pump pulses excite the cobalt layer at zero pump-probe delay time. The most striking feature of a pump-probe interferogram is the pronounced modulation of plasmonic interference fringes upon reflection of an acoustic pulse at the gold–air interface at a pump-probe delay time of t 0 =39 ps. The dynamics of the surface dielectric function in Fig. 1c (reconstructed from the pump-probe interferogram in Fig. 1b , see [14] for details) show that the acoustic modulation is due to the strong change of the real part of the dielectric function δε ′( t ). The monotonically increasing background signal in both δε ′( t ) and δε ″( t ) describes the slow temperature rise at the gold–air interface on a time scale of a few tens of picoseconds caused by heat diffusion in gold, an effect extensively discussed earlier [23] . Reconstruction of ultrashort acoustic strain pulses Information about the dielectric permittivity on an ultrafast time scale lets us now reconstruct the acoustic strain pulses at the gold–air interface. Assuming that the shape of the acoustic pulse does not change during acoustic reflection, that is, η ( z , t )= η ( t + z / c s )− η ( t − z / c s ), we obtain a more convenient expression for δε′ ( t ) 2| ε m | 2 δk sp ( t )/ k 0 : with η ( t )= η ( z =0, t − t 0 ) and τ skin = δ skin / c s . Taking the time-derivative dε ′/ dt leads to the following Fredholm integral equation of the second kind for the strain η ( t ): Whereas a solution of this integral equation for an arbitrary pulse is a difficult task, it may be simplified for an ultrashort acoustic pulse: as long as the duration of the acoustic pulse is shorter than the acoustic propagation time through the optical skin depth τ skin =3.8 ps, the first rapidly varying term in equation (3) dominates, and the numerical solution of Fredholm equation converges after a few iterations. In Fig. 2a we show the acoustic strain pulse obtained from the experimental data in Fig. 1c by solving equation (3). The inset in Fig. 2a illustrates the contributions from the two terms in equation (3). The first term given by the time-derivative dε ′/ d t determines the overall shape of the acoustic pulse. The shape is unaffected by small errors in the determination of the slowly varying background described by the second integral term. 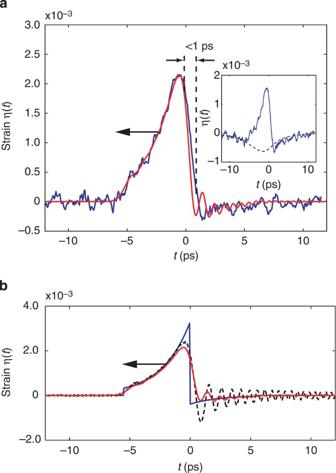Figure 2: Acoustic strain pulses at the gold–air interface. (a) The measured strain pulse (blue solid line) launched with a peak fluence of 7 mJ cm−2is in excellent agreement with the theoretical calculation (red solid line). The inset shows the two terms in equation (3): the first term (blue solid line) and the second term with opposite sign (dashed line). (b) Simulation of the strain pulses generated in cobalt (blue solid line) and after propagation through a 120-nm gold layer based on a linear model including dispersion (dashed line), as well as dispersion and SR (red solid line). The black arrow indicates the propagation direction of the acoustic pulses (compressional acoustic strain pulses have positive sign throughout the paper). Figure 2: Acoustic strain pulses at the gold–air interface. ( a ) The measured strain pulse (blue solid line) launched with a peak fluence of 7 mJ cm −2 is in excellent agreement with the theoretical calculation (red solid line). The inset shows the two terms in equation (3): the first term (blue solid line) and the second term with opposite sign (dashed line). ( b ) Simulation of the strain pulses generated in cobalt (blue solid line) and after propagation through a 120-nm gold layer based on a linear model including dispersion (dashed line), as well as dispersion and SR (red solid line). The black arrow indicates the propagation direction of the acoustic pulses (compressional acoustic strain pulses have positive sign throughout the paper). Full size image The retrieved acoustic pulse shape may be well approximated by simple linear modelling of acoustic propagation, as explained in detail in Fig. 2b . The initial strain pulse generated in the cobalt transducer is modelled with a simple exponential exp(−| t |/ τ 0 ) with τ 0 =2.5 ps, followed by a weak antisymmetric tail reflected from the cobalt–sapphire interface (acoustic reflectivity R =−0.11). Upon arrival at the gold–air interface, that is, after propagation through 120 nm gold, the acoustic strain pulse suffers from dispersion [24] . High-frequency components are left behind the pulse maximum, as observed in the high-frequency ripples in Fig. 2b . Moreover, the acoustic strain pulse experiences reflection at slightly different times due to nano-scale surface roughness (SR) at the gold–air interface. We used atomic force microscopy to quantify SR on all investigated samples. A typical SR of ~2 nm (root-mean-square) introduces a distribution of acoustic delay times within 600 fs (full-width half-maximum) and smears out the high-frequency ripples of the acoustic pulse ( Fig. 2b ). Excellent quantitative agreement between the experimental data and the linear model ( Fig. 2a ) taking into account acoustic dispersion and SR is achieved by setting the heat penetration depth in cobalt to 15 nm with km s −1 being the the speed of sound in (0001) direction in hcp-cobalt [25] . This value is ~1.5 times higher than the optical skin depth for 400 nm pump pulses in cobalt of 9.6 nm, in agreement with previously reported results for nickel films [5] . This similarity of nickel and cobalt is expected as the electron diffusion is particularly inefficient in Ni, Co and Fe because of their short electronic mean free paths [26] . The measured amplitude of the acoustic pulse 2 × 10 −3 agrees well with the strain due to thermal expansion of the laser-heated cobalt layer, estimated from the amount of absorbed pump energy. Possible contributions due to ultrafast magnetostriction [15] would lead to much smaller strain values below 1.5 × 10 −4 in cobalt [27] . It is important to note that the acoustic pulses entering the gold layer preserve their duration and exponential shape ~exp(− t / τ 0 ), but because of the 1.8 times smaller speed of sound in gold they become higher in strain and spatially contracted. Therefore, particularly high-strain amplitudes in gold should be feasible, in contrast to sapphire, where acoustic pulses become weaker for the same reason ( km s −1 in (0001) direction). Nonlinear acoustic propagation effects in gold In order to be able to work in the range of relatively high pump fluences, we had to use (for technical reasons) pump pulses at an optical wavelength of 800 nm, which were discriminated from probe pulses at the same wavelength by perpendicular polarization. Using this arrangement we performed a series of pump-power-dependent measurements with higher excitation fluence in two samples with an identical 35 nm thin cobalt transducer, but two different thicknesses of the gold layer, 120 and 220 nm. We clearly observe nonlinear reshaping of the acoustic pulses in both samples ( Fig. 3 ). Pulses with larger amplitude are moving faster. The reshaping is more pronounced in the thicker gold film. Both observations indicate the importance of nonlinear acoustic propagation in gold. 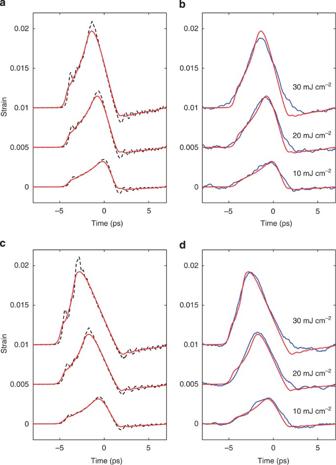Figure 3: Nonlinear reshaping of giant acoustic strain pulses in gold films. Measurements are made as a function of excitation fluence in 120 nm (a,b) and 220 nm (c,d) thick gold films deposited on a 35-nm thin cobalt transducer. (a,c) High-frequency components in the numerical solutions of the KdV equation (dashed line) are smeared out by SR (KdV+SR, red solid line). (b,d) Experimental curves (blue solid lines) demonstrate the nonlinear steepening of giant (up to 1 per cent) strain pulses, which becomes more pronounced for high excitation fluences and for thicker gold layers. The quantitative agreement with the KdV solutions (KdV+SR, red solid lines) is obtained by adjusting a single fit parameter, namely the 20 nm heat penetration depth in cobalt at 800 nm pump wavelength. No fit parameters were used to derive the experimental strain pulses. Curves for three different values of excitation fluence (10, 20 and 30 mJ cm−2) are vertically displaced for clarity. Our measurements are in excellent quantitative agreement with the solutions of the nonlinear Korteveg-de Vries (KdV) equation Figure 3: Nonlinear reshaping of giant acoustic strain pulses in gold films. Measurements are made as a function of excitation fluence in 120 nm ( a , b ) and 220 nm ( c , d ) thick gold films deposited on a 35-nm thin cobalt transducer. ( a , c ) High-frequency components in the numerical solutions of the KdV equation (dashed line) are smeared out by SR (KdV+SR, red solid line). ( b , d ) Experimental curves (blue solid lines) demonstrate the nonlinear steepening of giant (up to 1 per cent) strain pulses, which becomes more pronounced for high excitation fluences and for thicker gold layers. The quantitative agreement with the KdV solutions (KdV+SR, red solid lines) is obtained by adjusting a single fit parameter, namely the 20 nm heat penetration depth in cobalt at 800 nm pump wavelength. No fit parameters were used to derive the experimental strain pulses. Curves for three different values of excitation fluence (10, 20 and 30 mJ cm −2 ) are vertically displaced for clarity. Full size image These dynamics are governed by the interplay between the acoustic broadening due to phonon dispersion ω ( q )= c s q − γq 3 with γ =7.41 × 10 −18 m 3 s −1 and self-steepening and reshaping due to the elastic nonlinearity C 3 =−2.63 × 10 12 kg m −1 s −2 . See [20] for a definition of C 3 and [28] , [29] for linear and higher order elastic constants in gold; ρ =19.2 g cm −3 is the gold density. SR is again found to smear out possible high-frequency acoustic transients on a sub-picosecond time scale (compare KdV and KdV+SR in Fig. 3 ). Agreement between the nonlinear theory and the experiment is simply achieved by setting a single fit parameter, the initial heat penetration depth in cobalt δ heat =20 nm (corresponding to τ 0 =3.2 ps initial pulse duration). This value is again 50 per cent larger than the optical skin depth in cobalt of 13 nm. The quantitative agreement between theory and experiment for 120 and 220 nm thin gold layers clearly demonstrates that nonlinear reshaping is dominated by acoustic nonlinearities in gold. A possible dependence of the initial strain shape in cobalt on pump power obviously has a minor role. The amplitude of the acoustic strain reaches peak values η max =0.01, corresponding to a compressional stress GPa before acoustic reflection and negative −2.3 GPa tensile stress afterwards. At even higher pump powers, strain pulses up to 1.5 per cent were obtained but irreversible degradation of the samples was observed, consistent with elevating the temperature of the cobalt layer close to the melting point of 1,768 K. Control measurements at lower pump fluences confirmed that the nonlinear reshaping presented in Fig. 3 is fully reversible. Intrinsic damping of longitudinal phonons in gold caused by anharmonic phonon–phonon interactions [24] becomes increasingly important for frequencies exceeding 1 THz. However, in this frequency range and for our experimental geometry the effect of nano-scale SR entirely masks possible contributions due to phonon attenuation. Ultrafast acoustic pump-probe experiments in hybrid multilayer structures with a thicker gold layer and improved surface quality [30] may be performed to explore the mechanisms of terahertz phonon attenuation in metals. We have observed nonlinear reshaping of giant ultrashort acoustic pulses in gold at room temperature by applying femtosecond time-resolved surface plasmon interferometry. The ability to generate and quantify high-strain ultrashort acoustic pulses in hybrid metal/ferromagnet multilayer structures is most relevant for the emerging field of ultrafast magneto-acoustics [16] , [17] , [18] . The most prominent effects were obtained in the high-strain regime ( η max ~0.5%) using 200 nm nickel films [18] in which the nonlinear propagation effects are likely to be important. We envision using GPa acoustic pulses to switch magnetization in complex magnetostrictive materials such as Terfenol-D (ref. 31 ). This material is characterized by energy barriers between metastable magnetization directions in the MPa range and possesses an exceptionally high magnetostrictive coefficient of ~10 −3 , which is about two orders of magnitude higher than in Ni, Fe or Co (ref. 32 ). Theoretical estimates by Abrikosov show that our ultrashort GPa strain pulses can change the distribution function of electrons caused by phase-matched electron-phonon coupling resulting in the trapping of a small sub-ensemble of the electrons in the strain-induced deformation potential E Fermi η ~50 meV (ref. 33 ). This effect may stimulate novel applications of time-resolved photoelectron spectroscopy leading to the observation of transient strongly correlated electron-phonon states in metals on ultrafast time scales. Fabrication of gold–cobalt bilayers Hybrid acousto-plasmonic gold/cobalt/sapphire multilayer structures were manufactured by DC magnetron sputtering (base pressure: 2 × 10 −7 mbar; Ar sputter pressure: 10 −3 mbar) of a (111) gold layer on top of a hcp-cobalt film deposited on a (0001) sapphire substrate. Once loaded into the deposition chamber, sapphire substrates were outgassed for 30 min at 250 °C. Deposition of Co and Au layers was carried out also at 250 °C. First, a 35-nm thick Co layer was grown, then a (111)-textured gold layer with a thickness of 120–200 nm was deposited. Deposition rates were 12 nm min −1 for Au and 2 nm min −1 for Co. Nanometre SR was characterized by atomic force microscopy for each investigated sample. Tilted slit-groove microinterferometers Plasmonic slit-groove microinterferometers were milled into the multilayers with a 30-kV Ga + focussed ion beam. The slits were 100 nm wide and extended through both metal layers. The grooves were 200 nm wide and had a depth of 70 and 120 nm for gold thickness of 120 and 220 nm, respectively. The tilt angle between the slit and the groove was 10°. Optical measurements Time-resolved optical measurements were performed with an amplified femtosecond Ti:sapphire laser (Coherent RegA 250 kHz). The spatial period of the plasmonic interference pattern slightly varied depending on the angle of incidence of the probe beam, in agreement with predictions of geometrical optics. Technical details of the lock-in based scanning imaging set-up used to record plasmonic interferograms along the slit axes are given elsewhere in [14] . The Fourier method was used to extract phase and amplitude of plasmonic interference fringes. How to cite this article: Temnov, V.V. et al. Femtosecond nonlinear ultrasonics in gold probed with ultrashort surface plasmons. Nat. Commun. 4:1468 doi: 10.1038/ncomms2480 (2013).